Group A PP2Cs evolved in land plants as key regulators of intrinsic desiccation tolerance Vegetative desiccation tolerance is common in bryophytes, although this character has been lost in most vascular plants. The moss Physcomitrella patens survives complete desiccation if treated with abscisic acid (ABA). Group A protein phosphatases type 2C (PP2C) are negative regulators of abscisic acid signalling. Here we show that the elimination of Group A PP2C is sufficient to ensure P. patens survival to full desiccation, without ABA treatment, although its growth is severely hindered. Microarray analysis shows that the Group A PP2C-regulated genes exclusively overlap with genes exhibiting a high level of ABA induction. Group A PP2C disruption weakly affects ABA-activated kinase activity, indicating Group A PP2C action downstream of these kinases in the moss. We propose that Group A PP2C emerged in land plants to repress desiccation tolerance mechanisms, possibly facilitating plants propagation on land, whereas ABA releases the intrinsic desiccation tolerance from Group A PP2C regulation. Abscisic acid (ABA) has a major role in responses to water-restricted conditions in flowering plants, including stomatal closure, adaptation of vegetative tissues to drought, high salinity and low temperatures, and acquisition of desiccation tolerance and subsequent dormancy of seeds [1] , [2] . ABA has been also suggested to have a role in vegetative desiccation tolerance, a common feature of bryophytes (the basal land plants) but evolutionarily lost in vascular plants [3] , [4] , [5] . Protonemata of the model moss Physcomitrella patens are tolerant only to moderate water stress—that is, water loss up to around 90% of its fresh weight, or about −13 MPa by water potentials [6] —but not to complete desiccation in experimental conditions [6] , [7] . However, ABA pretreatment markedly increases their tolerance to complete desiccation [7] or equilibration to 13% relative humidity (−273 MPa) [6] . The inductive desiccation tolerance in vegetative tissues of the basal land plants, such as P. patens , suggests the hypothesis that acquisition of sensing and response mechanisms for ABA by their ancestors was critical for invasion of and adaptation to land, where water potentials were fluctuating continuously. Recent key studies in the vascular plant Arabidopsis provide evidence of a pivotal role of Group A protein phosphatases type 2C (PP2Cs) [8] , [9] , [10] , [11] , [12] in the ABA signalling pathway [13] . In the absence of ABA, Group A PP2Cs act through the physical interaction with subclass III of plant-specific SNF1-related protein kinases (SnRK2) and dephosphorylate the kinase activation loop, inhibiting ABA signalling transduction [14] , [15] , [16] , [17] , [18] , [19] . ABA binding to the receptor pyrabactin resistance 1-like (PYL) (also known as PYR or regulatory component of ABA receptor) [20] , [21] promotes the interaction between the receptor and the catalytic site of Group A PP2Cs [22] , [23] , leading to the inhibition of Group A PP2Cs and facilitating SnRK2 activation. It is evident that Group A PP2C is a central component in the induction of ABA signalling. Although genes for Group A PP2C are present only in the land plant lineage, they have expanded in number through land plant evolution. Group A PP2C of the flowering plant Arabidopsis consists of nine genes, whereas only two genes encode Group A PP2C in the moss P. patens . Therefore, the role of these two moss Group A PP2C genes could reflect ancestral functions. In fact, and as reported here, those two genes appear to be directly involved in ABA responses, including induced vegetative desiccation tolerance. Here we establish a null plant for Group A PP2C for the first time, taking advantage of efficient gene targeting in P. patens . Analysis of the null plant reveals that Group A PP2C represses the intrinsic feature of tolerance to desiccation, freezing and salinity, and promotes proliferation of the vegetative tissue. We further demonstrate that Group A PP2C exclusively regulates genes that exhibit a high level of ABA induction. In addition, our results show that Group A PP2C acts downstream of ABA-activated kinases in the moss. On the basis of these collective findings, we propose that Group A PP2C-mediated ABA signalling evolved in ancestral land plants to control pre-existing mechanisms for desiccation tolerance, facilitating rapid propagation on land. Role of Group A PP2C in growth and development We previously reported a loss-of-function analysis of PpABI1A single disruptants ( ppabi1a ) generated by gene targeting [24] . Either the wild-type (WT) or the ppabi1a plants were transformed with the PpABI1B -targeting construct to generate PpABI1B single disruptants ( ppabi1b ) or PpABI1 double disruptants ( ppabi1a / b ), respectively ( Supplementary Figs S1 and S2 ). We first analysed the effect of null expression of Group A PP2C on growth and development of P. patens under normal conditions. Previously, we reported that the ppabi1a single disruptant showed normal growth and development in the absence of exogenous ABA. As expected, the ppabi1b single disruptant also exhibited normal protonemal growth, as did WT and the ppabi1a single disruptant. However, the ppabi1a/b double disruptant showed a distinct phenotype in protonemal growth ( Fig. 1a–d ). The ppabi1a/b plants grew very slowly in a patchy fashion compared with the WT or both the single disruptants. Microscopic analysis of these filaments ( Fig. 1e,i ) revealed that each protonemal cell of the ppabi1a/b plants did not elongate like WT but differentiated into spherical brood cells, which are formed in the WT, only with exposure to exogenous ABA or to stress conditions [25] . Exogenous ABA has been known to prevent cytokinin-induced formation of buds that eventually develop into gametophores [26] . The protonemata of the ppabi1a/b , however, developed dwarf gametophores ( Fig. 1f,j ) at a frequency similar to that of WT. The gametophores of ppabi1a/b plants developed sporophytes indistinguishable from those of WT ( Fig. 1g,k ), and these spores also germinated ( Fig. 1h,l ). These results suggest that Group A PP2C is essential for proper growth, mainly for elongation of both protonemata and gametophores under non-stress conditions; however, it is not involved in developmental regulation, such as bud induction, gametophore development, embryogenesis or spore germination. 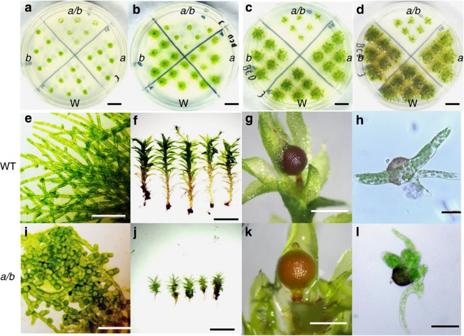Figure 1: Growth ofppabi1a/bdouble disruptants. Protonemal tissue was grown on BCD medium for (a) 1 week, (b) 2 weeks, (c) 4 weeks and (d) 2 months. W, wild type;a,ppabi1a;b,ppabi1b;a/b,ppabi1a/b. Magnified images of protonemal cells (e,i), gametophores grown on sterile peat pellets (f,j), sporophytes (g,k) and germinating spores (h,l). WT (e–h) andppabi1a/b(i–l). Scale bars ina–d, 1 cm;e, i, 200 μm;f,j, 5 mm;g,k, 0.5 mm; andh,l, 100 μm. Figure 1: Growth of ppabi1a/b double disruptants. Protonemal tissue was grown on BCD medium for ( a ) 1 week, ( b ) 2 weeks, ( c ) 4 weeks and ( d ) 2 months. W, wild type; a , ppabi1a ; b , ppabi1b ; a/b , ppabi1a/b . Magnified images of protonemal cells ( e , i ), gametophores grown on sterile peat pellets ( f , j ), sporophytes ( g , k ) and germinating spores ( h , l ). WT ( e – h ) and ppabi1a/b ( i – l ). Scale bars in a – d , 1 cm; e , i, 200 μm; f , j , 5 mm; g , k , 0.5 mm; and h , l , 100 μm. Full size image Role of Group A PP2C in stress responses To test the role of Group A PP2C in vegetative desiccation tolerance, protonemata were desiccated rapidly by exposure to an atmosphere of about −100 MPa (about 50% relative humidity) in a laminar flow cabinet for 24 h. This treatment resulted in almost complete removal of water (about 99% on a fresh weight basis) from the tissues of WT (as low as 0.056±0.002 g g dm −1 ; dm, dry matter) and ppabi1a/b plants (0.052±0.001 g g dm −1 ). It has been reported that only ABA-treated WT plants can survive this extremely dry condition [6] . According to these previous results, WT or the both single disruptants could not be recovered from desiccation stress after the treatment; here, however, ppabi1a/b plants survived and regrew without the assistance of exogenous ABA ( Fig. 2a,b ). The findings demonstrated that Group A PP2Cs repress the intrinsic desiccation tolerance of P. patens . 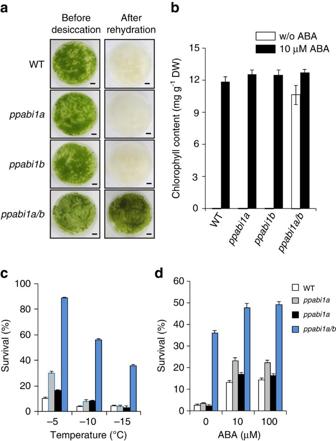Figure 2: Disruption ofPpABI1enhanced tolerance to desiccation and freezing in a gene dose–dependent manner. (a) One-week-old protonemata of WT and disruptants (ppabi1a,ppabi1bandppabi1a/b) were dried for 24 h, rehydrated with sterile distilled water and incubated for 2 weeks. Scale bars, 1 cm. (b) Chlorophyll content of WT and disruptants (ppabi1a, ppabi1bandppabi1a/b), treated with or without ABA (10 μM) for 24 h, was determined after desiccation assay. The values are mean±s.e. (n=3). (c) One-week-old protonemata of WT and disruptants (ppabi1a,ppabi1bandppabi1a/b) were frozen to −5 °C, −10 °C and −15 °C. Survival was determined by measuring the electrolyte leakage. (d) Protonemata cells were treated with indicated concentrations of ABA for 24 h and frozen to −15 °C. The values are mean±s.e. (n=3). DW, dry weight. Figure 2: Disruption of PpABI1 enhanced tolerance to desiccation and freezing in a gene dose–dependent manner. ( a ) One-week-old protonemata of WT and disruptants ( ppabi1a , ppabi1b and ppabi1a/b ) were dried for 24 h, rehydrated with sterile distilled water and incubated for 2 weeks. Scale bars, 1 cm. ( b ) Chlorophyll content of WT and disruptants ( ppabi1a, ppabi1b and ppabi1a/b ), treated with or without ABA (10 μM) for 24 h, was determined after desiccation assay. The values are mean±s.e. ( n =3). ( c ) One-week-old protonemata of WT and disruptants ( ppabi1a , ppabi1b and ppabi1a/b ) were frozen to −5 °C, −10 °C and −15 °C. Survival was determined by measuring the electrolyte leakage. ( d ) Protonemata cells were treated with indicated concentrations of ABA for 24 h and frozen to −15 °C. The values are mean±s.e. ( n =3). DW, dry weight. Full size image We also compared the freezing tolerance of the double-disruptant plants with that of WT or both single disruptants. Protonemal tissues of WT, both single disruptants, or double disruptants were exposed to subzero temperatures from −5 °C to −15 °C without ABA pretreatment, and the survival was calculated by measuring the electrolyte leakage ( Fig. 2c ). Protonemal cells of WT were not tolerant to freezing even at −5 °C. A slight but significant increase of freezing tolerance of the ppabi1a plants but not the ppabi1b plants was observed at −5 °C. On the other hand, the ppabi1a/b plants showed about 90% survival at −5 °C. The ppabi1a/b plants still showed about 40% survival even after freezing at −15 °C. At this temperature, WT protonemata treated even with 100 μM ABA for 24 h showed less than 20% survival ( Fig. 2d ). We further tested the tolerance of the ppabi1a/b plants to salinity. Protonemal colonies of WT or transgenic plants were challenged with a high concentration of NaCl for 5 days, then recovered on normal media for 7 days ( Supplementary Fig. S3 ). Growth of the ppabi1a/b plants was little affected by up to 450 mM NaCl. Taken together, these results suggest that Group A PP2C alleviates constitutive tolerances of protonemata to water-associated stresses in the absence of ABA. Late embryogenesis abundant (LEA) proteins are hydrophilic proteins that specifically accumulate in developing seeds or the water-stressed plant body, and are suggested to be involved in protection of cells from desiccation [27] . Because of this highly hydrophilic feature, LEA proteins are often boiling soluble [28] , [29] . When proteins from a protonemal crude extract were analysed, electrophoretic profiles were similar between WT and transgenic plants ( Supplementary Fig. S4 ); however, the accumulation profiles of boiling-soluble proteins were quite different ( Fig. 3a ). The ppabi1a/b plants accumulated boiling-soluble proteins in the absence of exogenously applied ABA, whereas accumulation of boiling-soluble proteins of WT or both single disruptants depended on ABA application. Exogenously applied ABA failed to enhance accumulation of boiling-soluble proteins in the ppabi1a/b plants. We further performed immunoblot experiments using specific antibodies against dehydrin (Group 2 LEA) or the LEA-like protein 17B9 (protein ID 171483), confirming the specific accumulation of LEA proteins in the ppabi1a/b plants but not in WT without ABA treatment ( Supplementary Fig. S5 ). We next performed analysis of the soluble sugar accumulation, because levels of soluble sugars associate with ABA-induced freezing tolerance in P. patens [30] . The ppabi1a/b plants accumulated considerable amounts of soluble sugars regardless of ABA application, whereas WT and both single disruptants increased accumulation of soluble sugars in response to ABA application ( Fig. 3b ). The analysis of soluble sugars showed constitutive accumulation of disaccharide as the major sugar and also detected trisaccharide with the same profile as that of ABA-treated WT ( Supplementary Fig. S6 ). These disaccharides and trisaccharides showing induced accumulation by ABA in WT were identified as sucrose and theanderose, respectively [30] . We also observed slight accumulation of additional sugar species in the ppabi1a/b plants, although their molecular characterizations are yet to be performed. These data suggest that the ppabi1a/b plants constitutively accumulate LEA proteins and soluble sugars at the maximum level even under standard growth conditions, which might be associated with extremely enhanced stress -tolerance. 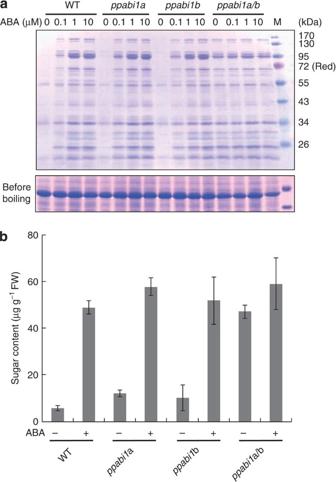Figure 3: Theppabi1a/bplants constitutively accumulate boiling-soluble proteins and soluble sugars. (a) Electrophoretic profiles of boiling-soluble proteins prepared from 1-week-old protonemata of WT and disruptants (ppabi1a,ppabi1bandppabi1a/b) treated with or without ABA for 24 h. Coomassie Brilliant Blue staining shows an equal amount of proteins subjected to boiling. M, molecular weight marker. (b) Soluble sugars extracted from WT and disruptants (ppabi1a,ppabi1bandppabi1a/b) treated with or without ABA (1 μM) for 24 h were analysed by anthrone-sulphuric acid assay. The values are mean±s.e. (n=3). FW, fresh weight. Figure 3: The ppabi1a/b plants constitutively accumulate boiling-soluble proteins and soluble sugars. ( a ) Electrophoretic profiles of boiling-soluble proteins prepared from 1-week-old protonemata of WT and disruptants ( ppabi1a , ppabi1b and ppabi1a/b ) treated with or without ABA for 24 h. Coomassie Brilliant Blue staining shows an equal amount of proteins subjected to boiling. M, molecular weight marker. ( b ) Soluble sugars extracted from WT and disruptants ( ppabi1a , ppabi1b and ppabi1a/b ) treated with or without ABA (1 μM) for 24 h were analysed by anthrone-sulphuric acid assay. The values are mean±s.e. ( n =3). FW, fresh weight. Full size image Role of Group A PP2C in global gene expression One open question is how globally Group A PP2C regulates ABA-responsive genes in land plants. To investigate the disruption effect of Group A PP2C on global gene expression, we performed microarray analysis of WT and transgenic plants using a custom Physcomitrella oligonucleotide microarray, which carries probes for 33,942 gene models of the Physcomitrella genome, version 1.1 on an Agilent platform. First, we compared expression profiles in the protonemata of the mutants with those of the WT in the absence of exogenous ABA ( Fig. 4a and Supplementary Data 1 ). The results showed that 354 genes, 131 genes and 873 genes were significantly upregulated (>2 fold) in ppabi1a , ppabi1b and ppabi1a/b , respectively. Approximately 95% and 62% of upregulated genes in ppabi1a and ppabi1b , respectively, were also upregulated in ppabi1a/b . Thus, PpABI1A and PpABI1B appear to be highly redundant, and PpABI1A has a more important role than PpABI1B in the ABA response of protonemata. 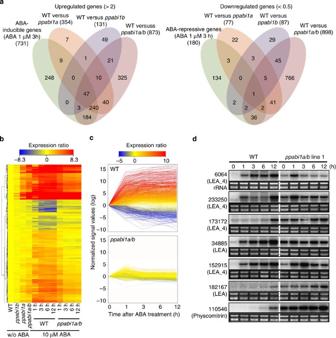Figure 4: Comparison of expression profiles of ABA-responsive genes between wild type andppabi1disruptants. (a) Venn diagrams show the number of upregulated genes (left) and downregulated genes (right) inppabi1disruptants compared with WT. (b) Hierarchical clustering of 911 ABA-responsive genes. Each gene is represented by a single row of coloured boxes. The colour represents the expression level of the gene. The range of induction and repression is shown from yellow to red and blue. (c) Comparison of expression patterns between ABA-responsive genes in WT andppabi1disruptants in time-dependent ABA treatment conditions. Each gene is represented by a coloured line. The colour represents the expression ratio of the gene at 12 h. (d) RNA analysis of ABA-inducible genes in theppabi1a/bplant. Protonemata were treated with 10 μM ABA for 0, 1, 3, 6 and 12 h, and isolated total RNA was subjected to RNA blot analysis for the indicated genes. Genes are indicated by Phypa IDs. For the full blots, seeSupplementary Fig. S7. Figure 4: Comparison of expression profiles of ABA-responsive genes between wild type and ppabi1 disruptants. ( a ) Venn diagrams show the number of upregulated genes (left) and downregulated genes (right) in ppabi1 disruptants compared with WT. ( b ) Hierarchical clustering of 911 ABA-responsive genes. Each gene is represented by a single row of coloured boxes. The colour represents the expression level of the gene. The range of induction and repression is shown from yellow to red and blue. ( c ) Comparison of expression patterns between ABA-responsive genes in WT and ppabi1 disruptants in time-dependent ABA treatment conditions. Each gene is represented by a coloured line. The colour represents the expression ratio of the gene at 12 h. ( d ) RNA analysis of ABA-inducible genes in the ppabi1a/b plant. Protonemata were treated with 10 μM ABA for 0, 1, 3, 6 and 12 h, and isolated total RNA was subjected to RNA blot analysis for the indicated genes. Genes are indicated by Phypa IDs. For the full blots, see Supplementary Fig. S7 . Full size image To investigate how many ABA-inducible genes are included in the 873 Group A PP2C-regulated genes, we selected 731 genes that were significantly induced (>2-fold) after 3 h of 1 μM ABA treatment in WT triplicate experiments. The number of ABA-inducible genes that were upregulated in the ppabi1a plants (296 genes) was much greater than in the ppabi1b plants (50 genes). Of note, the number of upregulated genes in the ppabi1a/b plants included 474 of the ABA-inducible genes. These results indicate that Group A PP2C regulates at least 65% of the ABA-inducible genes. Figure 4b shows a cluster analysis of the 911 ABA-responsive genes (731 inducible genes and 180 repressive genes in response to 1 μM ABA for 3 h) from the microarray data for WT plants and for the three ppabi1 transgenics. In the absence of exogenous ABA, the ppabi1a/b plants showed the closest expression profile to that of ABA-treated WT. We also compared the expression patterns of the 911 ABA-regulated genes after ABA treatment ( Fig. 4c ). Compared with the WT, the response of these genes in the ppabi1a/b plants to exogenous ABA was greatly reduced, indicating that expression of ABA-regulated genes in the ppabi1a/b plants is mostly saturated without ABA application. We also confirmed the expression profile of several ABA-inducible genes by RNA blot analysis ( Fig. 4d and Supplementary Fig. S7 ). Consistent with the results of the microarray analysis, the ppabi1a/b plants accumulated the transcripts of these ABA-inducible genes in the absence of exogenous ABA, and exogenously applied ABA affected the expression levels only slightly, although some genes still showed significant transient activation by ABA. We found that considerable numbers of ABA-inducible genes (>10-fold) were under the regulation of Group A PP2C ( Supplementary Fig. S8 ). To understand the impact of the Group A PP2C-mediated gene regulation system on genome-wide ABA response, we traced the time course of whole genes in WT that gave sufficient signal intensity for investigation (14,721 genes) and also the time course of the 1,771 Group A PP2C-regulated genes (873 upregulated genes and 898 downregulated genes) ( Fig. 5a,b ). When the expression profiles of Group A PP2C-regulated genes were removed from the whole gene expression profile ( Fig. 5c ), genes that were highly induced by ABA had almost disappeared. These results indicate that Group A PP2C is essential for the genome-wide induction system of gene expression in response to ABA. To investigate the main target of Group A PP2C in P. patens , we selected the top 100 genes that showed a high level of induction in ppabi1a/b plants in the absence of ABA. Although most of the genes were categorized as ‘unknown function’, it should be noted that 13 LEA genes were included ( Supplementary Data 2 ). To determine how many LEA genes are under the regulation of Group A PP2C, we selected putative LEA genes from P. patens genome databases and investigated the ABA responses ( Supplementary Data 3 ). As a result, 77 genes were considered to encode LEA proteins. Among these genes, 67 were included in our custom array chip. A total of 42 of 67 putative LEA genes were upregulated (>2-fold) by exogenous ABA in WT; the remaining genes were not influenced or downregulated by exogenous ABA in WT. In the absence of exogenous ABA, the ppabi1a/b plants constitutively upregulated 39 out of 42 ‘ABA upregulated’ LEA genes, including dehydrin genes and 17B9 , the gene products of which were also detected by immunoblot analysis ( Supplementary Fig. S5 ). These data suggest that expression of LEA genes is strongly associated with Group A PP2C-mediated ABA signalling and with tolerances to desiccation, freezing and salinity in the moss. 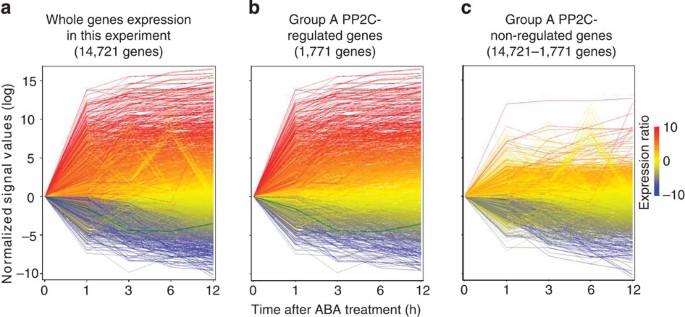Figure 5: Comparison of expression patterns between Group A PP2C-regulated and non-regulated genes in ABA treatment conditions. (a) Expression patterns of whole expressed genes (left), (b) Group A PP2C-regulated genes (centre) and (c) Group A PP2C non-regulated genes (right) in ABA-treated wild-type plants are shown as a profile plot. Each gene is represented by a coloured line. The colour represents the expression ratio of the gene at 12 h. Figure 5: Comparison of expression patterns between Group A PP2C-regulated and non-regulated genes in ABA treatment conditions. ( a ) Expression patterns of whole expressed genes (left), ( b ) Group A PP2C-regulated genes (centre) and ( c ) Group A PP2C non-regulated genes (right) in ABA-treated wild-type plants are shown as a profile plot. Each gene is represented by a coloured line. The colour represents the expression ratio of the gene at 12 h. Full size image Activity of ABA-activated protein kinases in ppabi1 plants ABA induces activity of specific protein kinases in angiosperms. In Arabidopsis, ABA-activated kinase activity is lost in a triple disruptant of subclass III SnRK2s, suggesting that subclass III SnRK2s are the major kinases for ABA-induced phosphorylation [16] , [17] , [18] , [19] . According to the current model of initiation of ABA signalling in which Group A PP2C negatively regulates activity of SnRK2, ppabi1a/b plants were expected to show constitutive activation of ABA-activated kinase regardless of ABA application. We compared the activity of ABA-activated kinases between WT and the three ppabi1 transgenics using an in-gel phosphorylation assay with histone as a substrate ( Fig. 6 ). This method has been successfully employed to detect SnRK2 activity in angiosperms [14] , [31] , [32] . As observed in angiosperms, upon ABA application, P. patens also rapidly increased kinase activity, detected as one heavy band corresponding to the expected molecular weight (about 40 KDa) of SnRK2s from P. patens , whose genome encodes only subclass III SnRK2 (ref. 33 ). To our surprise, this ABA-activated kinase activity occurred only slightly in ppabi1a/b plants in the absence of exogenous ABA and was markedly activated by ABA application followed by subsequent reduction of the kinase activity. This result indicates that Group A PP2C is not the major factor regulating ABA-activated kinases and instead acts downstream of the kinases. Our data also suggest the presence of another mechanism for the regulation of kinase activity by ABA. 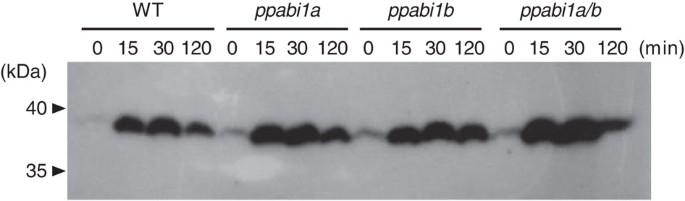Figure 6: Effect ofPpABI1disruption on ABA-activated protein kinases. One-week-old protonemata of WT and disruptants (ppabi1a,ppabi1bandppabi1a/b) were treated with 10 μM ABA for 0, 15, 30 or 120 min and subjected to in-gel phosphorylation assay using histone IIIS as a substrate. Figure 6: Effect of PpABI1 disruption on ABA-activated protein kinases. One-week-old protonemata of WT and disruptants ( ppabi1a , ppabi1b and ppabi1a/b ) were treated with 10 μM ABA for 0, 15, 30 or 120 min and subjected to in-gel phosphorylation assay using histone IIIS as a substrate. Full size image We investigated the subcellular localization of the green fluorescent protein (GFP)–PpABI1A fusion protein in P. patens protonemal cells. The GFP–PpABI1A fusion protein predominantly localized to the nucleus, whereas the Arabidopsis GFP–ABI1 fusion protein was found in both the cytosol and the nucleus, as has been reported [34] ( Supplementary Fig. S9 ). These data indicate that Group A PP2C mainly functions in the nucleus in P. patens . Evolution of the ABA core components PYL/PP2C/SnRK2 in land plants must have had a key role in enabling adaptation to the terrestrial environment. ABA has been shown to be responsible for stomatal closures and seed desiccation tolerance in angiosperms, both of which are related to adaptation to water-stress conditions. OPEN STOMATA1 , a causal gene of an Arabidopsis mutant that has defects in stomatal closure, encodes subclass III SnRK2.6 (ref. 15 ). Recently, SnRK2s from the lycophyte Selaginella uncinata and the moss P. patens have been shown to rescue the Arabidopsis ost1 mutant [35] , [36] , suggesting an evolutionarily conserved function of SnRK2 in the machinery of stomatal closure among land plants. However, what remains a matter of debate is when land plants acquired the ABA-dependent closure system of the stomatal aperture in their evolutionary history [35] , [36] , [37] , [38] . Stomata are widely distributed among land plants, except liverworts, indicating that the epidermal apparatus evolved after the separation of liverworts and mosses from a common ancestor more than 400 million years ago. In contrast, ABA signalling that involves Group A PP2C can be found in liverworts [39] , suggesting that the ABA core components evolved to regulate physiological aspects other than stomata control. Vegetative desiccation tolerance is considered to have been a key component for successful land colonization in the evolution of green plants [40] , and ABA has been shown to regulate this physiological response in bryophytes by a mechanism similar to that of seed desiccation tolerance [7] . In this study, we demonstrated that elimination of Group A PP2C is sufficient to confer desiccation tolerance on P. patens without any treatment, that is, without exogenous ABA. One might speculate that these phenotypes result from the increased endogenous ABA in the ppabi1a/b plants. However, we observed a marked activation of ABA-activated kinases after ABA treatment, such as that of the WT. Moreover, we found no significant expression changes in ppabi1a/b plants of genes encoding 9-cis-epoxycarotenoid dioxygenase or zeaxanthin epoxidase, key enzymes in the ABA biosynthesis pathway [41] . These data indicate that desiccation tolerance of the ppabi1a/b plants was not the result of the overaccumulation of endogenous ABA. Taken together, the evidence shows that the default status of P. patens protonemata is desiccation tolerance, but that Group A PP2C represses this intrinsic feature in the absence of stresses, possibly to prioritize rapid propagation on land. In fact, growth of P. patens lacking Group A PP2C was severely retarded. From this point of view, ABA is simply acting to release the intrinsic ability of desiccation tolerance from Group A PP2C regulation. Elimination of Group A PP2C resulted in activation (>2-fold) of 873 genes as well as repression (<0.5-fold) of 898 genes; thus, Group A PP2C regulates expression of at least 1,771 genes. These genes account for about 4.6% of the total P. patens 38,357 gene models ( www.cosmoss.org database, Ver. 1.6). Expression profiles of P. patens genes that are not regulated by Group A PP2C specifically lacked a high level of ABA induction. We also showed that most of the ABA upregulated LEA genes are under the regulation of Group A PP2C in P. patens . These data agree well with the fact that the ppabi1a/b plants constitutively accumulated boiling-soluble proteins, which is a characteristic feature of LEA proteins. The implication is that expression of LEA genes is strongly associated with Group A PP2C-mediated ABA signalling and with tolerances to desiccation, freezing and salinity in the moss. LEA proteins are widespread in the plant kingdom, from algae to seed plants [33] , [42] . These transcripts accumulate in response to water-stress conditions even in algae. Although ABA can be found in algae, these organisms do not possess core components of ABA signalling, including Group A PP2Cs, and have very low sensitivity to exogenous ABA [33] . Stress-induced expression of LEA genes in algae might be mediated via different mechanisms from land plants. Our findings suggest that the core components of ABA signalling and regulation of LEA gene expression in response to water-related stresses coevolved in ancestral land plants. To our surprise, ABA-activated kinases in ppabi1a/b plants were only slightly activated but not hyperactivated in the absence of ABA, and were considerably activated by ABA application, followed by rapid reduction. This result raises several issues regarding the proposed role of Group A PP2C. First, Group A PP2Cs may be partly involved but does not have a major role in the regulation in P. patens of ABA-activated kinases, probably SnRK2s. Thus, the default status of ABA-activated kinases is ‘off’, and there is an as-yet-unknown system to activate the kinases. It has been suggested that SnRK2 activity is mainly regulated by reversible phosphorylation/dephosphorylation of a conserved Ser (S175 in SnRK2.6) in the intramolecular domain, called an activation loop [43] , [44] . In the well-established model in angiosperms, Group A PP2C dephosphorylates the conserved Ser and binds to the kinase domain to block the access of substrates in the absence of ABA [45] . Upon ABA perception, PYL-related ABA receptors bind to the catalytic site of Group A PP2C [22] , [23] , [46] that inhibits their enzymatic activity. This inhibition in turn allows SnRK2 to become partially active through the structural stabilization of the kinase domain, enabling autophosphorylation of the activation loop [47] . In P. patens , removal of Group A PP2C was not sufficient to fully activate the ABA-activated kinases, strongly suggesting PP2C-independent mechanisms for their ABA activation. Phosphorylation of SnRK2 by osmostress and ABA also involves unidentified staurosporine-insensitive upstream kinases in Arabidopsis [43] . This type of kinase might have a major role in activation of ABA-activated kinases in the basal land plants. We speculate that a strong association between SnRK2 and Group A PP2C might have developed in the vascular plant lineage after separation from the bryophytes. In fact, the ABA box, which is located at the carboxy-terminal of Arabidopsis SnRK2 and is responsible for the interaction with Group A PP2Cs [45] , [48] , is less conserved in the four subclass III SnRK2s encoded in the P. patens genome ( Supplementary Fig. S10 ). The second issue related to the kinase activation results in our ppabi1a/b plants is that even in the absence of Group A PP2C, negative feedback regulation of ABA-activated kinases was observed. Accumulation of Group A PP2C mRNA is increased after ABA treatment [11] . This response was considered to be the negative feedback regulation of ABA signalling. However, again, our results indicate that Group A PP2C is not a major factor in the negative feedback system for repressing ABA-activated kinases and that there must be another protein phosphatase responsible for their inactivation. Several reports describe proteins that can interact with Group A PP2C, including SnRK3-type protein kinase SOS2 (ref. 49 ), a potassium channel AKT3 (ref. 50 ), ATHB6 transcription factor [51] and SWI3B chromatin remodelling factor [52] . Our data demonstrate that Group A PP2C negatively regulates a signalling pathway downstream of ABA-activated kinases, confirming that Group A PP2C acts at different layers of ABA signalling. As the ppabi1a/b plants showed constitutive activation of the ABA-signalling pathway that is not necessarily related to the activity of ABA-activated kinases, the target of Group A PP2C must be a key component for acquisition of desiccation tolerance. As intensive nuclear localization of the GFP–PpABI1A fusion protein was observed here in transiently transformed protonemal cells regardless of ABA application, the major target of Group A PP2C must be present in the nucleus. We have developed a working model for the evolution of Group A PP2C-mediated ABA signalling in land plants ( Fig. 7 ). Before the emergence of Group A PP2Cs, activation of the pathway for vegetative desiccation tolerance might have been a default status in ancestral land plants, as observed in ppabi1a/b plants. In the next evolutionary step, the ancestor of bryophytes recruited Group A PP2Cs as key regulators to control this pre-existing desiccation tolerance pathway downstream of the kinases in an ABA-dependent manner, with newly evolved ABA receptors, PYLs, for better growth to survive on land. Later during their evolution, the ancestor of seed plants acquired novel SnRK2 substrates, such as ABI5-related bZIPs [53] , [54] and SLAC1, a critical anion channel for stomatal closure [55] , [56] , possibly leading to the emergence of distinct ABA-signalling branches to control seed germination and stomatal closures. The development of a strong interaction between SnRK2 and PP2C would have enabled tight regulation of SnRK2 by PP2C, which might be necessary for control of the increased numbers of downstream signalling pathways of SnRK2. 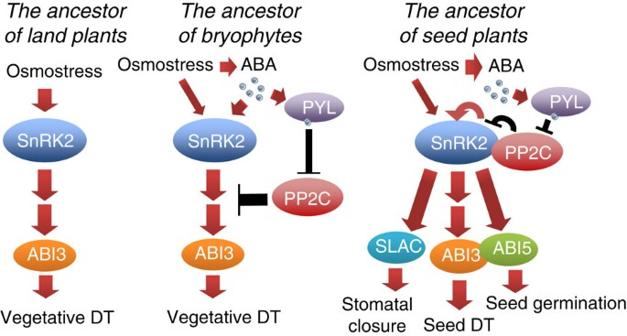Figure 7: Evolutionary model of Group A PP2C–mediated ABA signalling. The ancestor of bryophytes (middle) recruited PP2C to control the pre-existing pathway for vegetative desiccation tolerance (DT) (left) in an ABA-dependent manner. Note the PP2C action downstream of SnRK2. The ancestor of seed plants (right) developed tight regulation of SnRK2 by PP2C, which enabled integrated regulation of an increased number of signalling pathways downstream of SnRK2. Figure 7: Evolutionary model of Group A PP2C–mediated ABA signalling. The ancestor of bryophytes (middle) recruited PP2C to control the pre-existing pathway for vegetative desiccation tolerance (DT) (left) in an ABA-dependent manner. Note the PP2C action downstream of SnRK2. The ancestor of seed plants (right) developed tight regulation of SnRK2 by PP2C, which enabled integrated regulation of an increased number of signalling pathways downstream of SnRK2. Full size image Plant materials P. patens subspecies patens (Gransden) was the WT strain. Protonemal tissue was grown on BCDAT medium at 25 °C under continuous light (50–80 μmol m −2 s −1 ) [24] . The gametophores were induced on sterile peat pellets (Jiffy-7, Sakata Seed, Japan) in a plant culture box by culturing at 25 °C under continuous light for 1–1.5 months. For induction of sporophytes, gametophore cultures were transferred to 15°C under 8 h light/16 h dark conditions. Targeting construct for PpABI1B To create the PpABI1B targeting construct, the upstream (3,067 bp) and downstream regions (3,053 bp) of the open-reading frame were amplified by PCR using KOD Plus (Toyobo, Japan) with the following primer pairs: 5′-CCGCATTTGCCTAAGACTTC-3′/5′-GAATTTCCATCCTGCGACGC-3′ and 5′-ATAGGTAACCCGTGGATGGT-3′/5′-AGAGCTACATGCATTTCAAG-3′ for upstream and downstream regions of PpABI1B , respectively. The amplified fragments were verified by sequencing and cloned into both ends of the hygromycin resistance cassette in pBlueScript KS+ (Agilent Technologies, USA). Preparation of protoplasts from PpABI1A single-disruptant plants ( ppabi1a ) and the transformation were carried out by polyethylene glycol-mediated method [24] and 25 μg ml −1 hygromycin was used for screening of transformants. Genomic PCR Genomic DNA was isolated using PhytoPure (GE Healthcare, UK) with an additional RNase treatment. To check homologous recombination at the 5′- and 3′-flanking regions of the PpABI1B genomic locus, PCR was performed using primer set A for the 5′-recombination and primer set B for the 3′-recombination. The absence of the PpABI1B genomic region was confirmed by PCR using KOD FX (Toyobo, Japan) with primer set C. The PCR condition was 30 cycles at 98 °C for 10 s, 45 °C for 30 s and 68 °C for 15 s. The lack of transcripts corresponding to PpABI1A and/or PpABI1B in the ppabi1b and ppabi1a/b plants was confirmed in microarray analysis (see below). The primer sets are described in Supplementary Table S1 . Southern blot analysis The genomic DNA of the ppabi1a/b plants was extracted using PhytoPure (GE Healthcare, UK) with an additional RNase treatment. The probe for hygromycin was amplified using a PCR DIG Probe Synthesis Kit (Roche Applied Science, Germany) with PCR and the following primers: 5′-CCGGAGATTACAATGGACGA-3′/5′-TTCTTCCACGAAGCTCCTCG-3′. Insertion of the PpABI1B disruption construct was analysed using 2 μg of genomic DNA digested with Nde I. Digested DNA was separated on 0.6% agarose gels and transferred to nylon filters (Hybond-N+, GE Healthcare). The membrane was hybridized with DIG-labelled probes in DIG Easy Hyb buffer (Roche Applied Science) at 41 °C overnight. After washing, the membrane was treated once with blocking buffer for 1 h at room temperature. The membrane was reacted with Anti-Dig (Roche Applied Science) for 1 h at room temperature. Detection was carried out with CDP-Star (Roche Applied Science) for 5 min at room temperature in the dark. The signal was detected by ChemiDoc XRS Plus (Bio-Rad Laboratories, USA). RNA blot analysis Total RNAs were extracted from protonemal tissues using the RNeasy plant mini Kit (QIAGEN, USA). Ten micrograms of total RNA was separated by a formaldehyde-denaturing agarose gel and transferred onto a nylon membrane. Probes were generated by PCR of complementary DNA prepared from ABA-treated WT plants. The primer sets are described in Supplementary Data 4 . PCR fragments were purified using the Gel Extraction kit (QIAGEN, USA). Hybridization with 32 P-labelled DNA probes was carried out [24] . BAStaion 2500 (Fuji Film, Japan) was used for visualization of the blots. Protein analyses Protonemal cells were homogenized and extracted with 50 mM Tris (pH 7.5), 100 mM NaCl, 0.1% Triton X-100, 0.1 mM EDTA, 2 mM dithiothreitol (DTT) and 1 mM phenylmethylsulphonyl fluoride on ice. After centrifugation at 14,000 g for 10 min at 4 °C, supernatants were used as crude fractions. The proteins in the crude fractions, adjusted to equal concentrations, were boiled for 10 min, and insoluble pellets were removed by centrifugation at 14,000 g for 10 min at 4 °C. These soluble fractions were used as boiling-soluble proteins. The boiling-soluble proteins corresponding to 20 μg of crude proteins were used for gel electrophoresis. The crude proteins and boiling-soluble proteins were separated on 12% (w/v) SDS–polyacrylamide gels. After electrophoresis, proteins were stained using Coomassie Brilliant Blue. Soluble sugar measurement Protonema tissues were homogenized at 0 °C in 5 ml of EtOH–H 2 O (4:1). The homogenate was centrifuged at 14,000 g for 5 min at 4 °C, and the supernatant was recovered. After evaporation of ethanol, the samples were dissolved in distilled H 2 O (0.5 ml) and centrifuged at 14,000 g for 5 min at 4 °C to remove any debris. Soluble sugars in the supernatant were quantified by the anthrone-sulphuric acid assay using glucose as a standard [57] . Desiccation assay Protonemal tissues grown for 7 days on cellophane-layered BCDAT medium, treated with or without ABA for 24 h, were transferred to an empty Petri dish and desiccated inside a laminar flow hood for 24 h. The desiccated tissues were rehydrated with 5 ml of sterile water. These rehydrated tissues were then incubated under the standard growth conditions described above for 2 weeks. Measurement of water content was calculated as the difference between the fresh weight and the oven dry weight, divided by the oven dry weight [6] . Measurement of chlorophyll content The chlorophyll of the homogenized protonemal tissue was extracted with 10 ml of 80% (v/v) acetone. To remove cell debris, the samples were centrifuged for 5 min at 9,000 g . Supernatants were measured at wavelengths of 645 and 663 nm for the chlorophyll quantification. After measurement, the supernatant was dried up in the initial tube at room temperature until a stable dry weight of each sample was obtained. The total chlorophyll was calculated as follows: mg chlorophyll per g dry weight=[(A 663 )(0.00802)+(A 645 )(0.0202)] × 50/dry weight. Measurement of freezing tolerance Freezing tolerance was determined by measurement of electrolyte leakage after equilibrium freezing to various subzero temperatures. The amount of electrolyte leakage from the freeze-thawed tissues (Eft) was then determined by measuring electroconductivity. After the measurement, the tubes containing the samples were boiled for 10 min, and the amount of electrolytes after boiling (Eb) was determined. Survival of the cells was represented as the Eft/Eb ratio (%). Transcriptome analysis Microarray analysis was performed using a P. patens custom oligonucleotide microarray. Gene sequences used for oligonucleotide probe development were obtained from P. patens subsp. patens version 1.1 genome annotation [58] . For 35,938 gene models, 60-mer oligonucleotide probes were designed from the 3′-region of the sequence in consideration of Tm value, CG content, matching against expressed sequence tag and gene specificity; finally, 33,942 gene-specific probes were mounted in an Agilent format microarray. Total RNA was extracted from ABA-treated protonemal tissues of WT plants and from the three ppabi1 transgenics. For definition of significant ABA-regulated genes in WT and identification of differentially expressed genes in the three ppabi1 transgenics, three biological replicate samples were analysed. The microarray experiments were performed using the Agilent one-colour method according to the manufacturer’s instructions. Spot signal values were calculated by Feature Extraction ver. 9.1 software (Agilent Technologies). Digitalized signal values were imported into GeneSpring GX software (Agilent Technologies) and normalized to shift to the 75th percentile. Quality control was carried out with a filter for intensity value; probes with intensity values less than 500 in any experiments were removed. After filtering for intensity value, a total of 14,721 probes were subjected to further analysis. Fold-change analysis was performed on triple replicate samples to determine ABA-regulated genes and PpABI1-regulated genes. A twofold expression cut-off was considered to determine upregulated and downregulated genes ( Supplementary Data 1 ). The false discovery rate for the analysis was 0.05. In-gel phosphorylation assay One-week-old protonemata were treated with 10 μM ABA. Tissues were crushed by a mortar in liquid nitrogen and homogenized in extraction buffer containing 50 mM HEPES pH 7.5, 5 mM EDTA, 5 mM EGTA, 25 mM NaF, 2 mM DTT, 1 mM Na 3 VO 4 , 2 mg ml −1 leupeptin, 2 mg ml −1 pepstatin A, 2 mM phenylmethylsulphonyl fluoride, 50 mM β-glycerophosphate and 20% glycerol. Equal amounts of total soluble proteins were electrophoresed in 10% SDS–polyacrylamide gel to which 0.5% (w/v) histone IIIS (Sigma, MO, USA) had been added. After denaturation and renaturation procedures, the kinase activity was detected by incubation with 50 μM γ- 32 P-labelled ATP in a buffer containing 40 mM Hepes–KOH (pH 7.5), 5 mM MgCl 2 , 2 mM DTT and 0.1 mM EGTA, followed by washing and autoradiography [59] . Accession codes: The microarray data were deposited to NCBI Gene Expression Omnibus (accession GSE37694 ). How to cite this article : Komatsu, K. et al. Group A PP2Cs evolved in land plants as key regulators of intrinsic desiccation tolerance. Nat. Commun. 4:2219 doi: 10.1038/ncomms3219 (2013)